Realization of a three-dimensional spin–anisotropic harmonic honeycomb iridate Spin and orbital quantum numbers play a key role in the physics of Mott insulators, but in most systems they are connected only indirectly—via the Pauli exclusion principle and the Coulomb interaction. Iridium-based oxides (iridates) introduce strong spin–orbit coupling directly, such that these numbers become entwined together and the Mott physics attains a strong orbital character. In the layered honeycomb iridates this is thought to generate highly spin–anisotropic magnetic interactions, coupling the spin to a given spatial direction of exchange and leading to strongly frustrated magnetism. Here we report a new iridate structure that has the same local connectivity as the layered honeycomb and exhibits striking evidence for highly spin–anisotropic exchange. The basic structural units of this material suggest that a new family of three-dimensional structures could exist, the ‘harmonic honeycomb’ iridates, of which the present compound is the first example. Quantum spin systems are characterized by a spin that is decoupled from the crystal lattice, in contrast to Ising-like spin systems that often apply to higher spin states. In the Heisenberg model describing spin-isotropic exchange between neigbouring spins, spatial anisotropies of the exchange suppress long-range order [1] , but do not lead to anisotropy of the magnetic susceptibility. Striking examples of this are quasi-one- and two-dimensional systems, where the exchange differs by orders of magnitude for neighbours along distinct crystallographic directions [2] , [3] . The spin–orbit interaction introduces magnetic anisotropy by coupling the spin to the symmetry of the local orbital environment. Although in spin-½ systems the crystal field does not introduce single-ion anisotropy (due to Kramer’s protection of the spin-½ doublet), it can—via spin–orbit—introduce spin-anisotropies in the g -factor and in the exchange interactions. The strength of the spin–orbit coupling varies by orders of magnitude between the 3 d and 5 d transition metals. In the former, quenching of the orbital moment decouples the orbital wavefunction from the spin, giving a g -factor anisotropy that is typically small and an even smaller spin-anisotropy. For example, spin-½ copper in a tetragonal crystal field has a g -factor anisotropy of order 10%, whereas the spin-anisotropy of exchange is of the order of 1% (ref. 3 ). The stronger spin–orbit coupling of the 5 d transition metals is known to give rise to larger magnetic anisotropies. In materials with edge-shared IrO 6 octahedra, spin-anisotropy of the exchange between neighbouring effective spin-½ states is enhanced by the interference of the two exchange paths across the planar Ir–O 2 –Ir bond. Jackeli and Khaliullin (JK) [4] suggested that in the honeycomb iridates this may lead to extreme spin-anisotropy of the exchange coupling, where in the limiting case, the only non-vanishing interaction is for the spin component normal to the Ir–O 2 –Ir plane [4] , [5] , [6] . In the honeycomb lattice, such an interaction couples different orthogonal spin components for the three nearest neighbours; no single exchange direction can be simultaneously satisfied, leading to strong frustration. It is the possibility of engineering spin-anisotropy coupled to spatial exchange pathways that has spurred intense scientific research, particularly in connection to the search for quantum spin-liquids [4] , [5] , [6] , [7] . However, whether the spin–anisotropic exchange interaction that is coupled to the Ir–O 2 –Ir bonding plane is realized in such materials remains an intense subject of scientific debate [6] , [8] , [9] , [10] , highlighting the need for the discovery of new materials with related structures and strong anisotropic exchange interactions. We have synthesized single crystals of a new polytype of Li 2 IrO 3 in which we reveal the effect of the spin-anisotropy of exchange from the temperature dependence of the anisotropic magnetic susceptibility. Crystal structure Single crystals of Li 2 IrO 3 were synthesized as described in Methods. As shown in Fig. 1a , the crystals are clearly faceted and typically around 100 × 100 × 200 μm 3 in size. In contrast to the monoclinic structure of the layered iridate, we find that these materials are orthorhombic and belong to the non-symmorphic space group Cccm , with lattice parameters a =5.9119(3) Å, b =8.4461(5) Å and c =17.8363(10) Å (see Supplementary Discussion and Supplementary Data 1 for details of the crystallography). The structure (shown in Fig. 1b,c ) contains two interlaced honeycomb planes, the orientation of which alternate along the c axis. 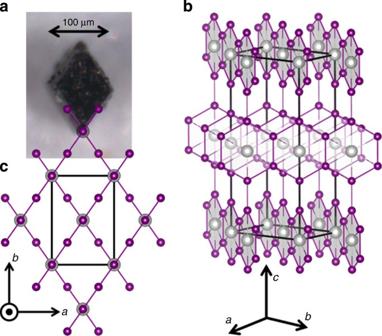Figure 1: Single crystal of ‹1›-Li2IrO3and the Ir lattice structure. (a) Single crystal oriented to be parallel to the crystallographic axes shown in (c), (b) three-dimensional view and (c) projection in theabplane. Inb, the grey shading emphasizes the Ir (purple balls) honeycomb rows that run parallel to thea±bdiagonals, alternating upon moving along thecaxis. For simplicity only Li ions (grey balls) located in the center of Ir honeycombs are shown. Inb,cthe rectangular box indicates the unit cell. Comparingawithcwe note that the∼70° angle between honeycomb rows is evident in the crystalline morphology. The X-ray refinement (see Supplementary Discussion ; Supplementary Figs 1–4 ; Supplementary Table 1 ) is consistent with fully stoichiometric Li 2 IrO 3 . In this case the Ir oxidation state is Ir 4+ (5 d 5 ), fixing the effective Ir local moment J eff =½, which is consistent with the magnetic properties of our crystals (see Fig. 2 ). In addition, highly sensitive single-crystal susceptibility and torque measurements (see below) observe sharp anomalies at the transition to magnetic order, with no measurable variability in this transition temperature between many crystals measured, indicating that the observed magnetic order is well formed and intrinsic to the crystals. This suggests that if present, Li vacancy disorder is small, because such vacancies will to lead non-magnetic Ir 5+ 5 d 4 (ref. 11 ), whose presence is expected to give rise to spin-glass behaviour [12] , which we do not observe. Taken together, our experiments indicate that our crystals are representative of the high-purity, stoichiometric limit. We denote the crystal structure ‹1›-Li 2 IrO 3 , where ‹1› refers to the single, complete oneycomb row. Figure 1: Single crystal of ‹1›-Li 2 IrO 3 and the Ir lattice structure. ( a ) Single crystal oriented to be parallel to the crystallographic axes shown in ( c ), ( b ) three-dimensional view and ( c ) projection in the ab plane. In b , the grey shading emphasizes the Ir (purple balls) honeycomb rows that run parallel to the a ± b diagonals, alternating upon moving along the c axis. For simplicity only Li ions (grey balls) located in the center of Ir honeycombs are shown. In b , c the rectangular box indicates the unit cell. Comparing a with c we note that the ∼ 70° angle between honeycomb rows is evident in the crystalline morphology. 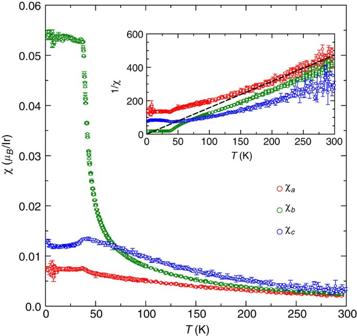Figure 2: The temperature dependence of the single-crystal magnetic susceptibility along the three principal crystalline directions. The inset shows 1/χfor all three axesχa,χbandχc. The dashed line indicates the slope of the inverse Curie–Weiss susceptibility for a paramagnet with effective moment ofμeff=1.6 μB, close to that expected of an IrJeff=½ state if theg-factor anisotropy is ignored. All three components of susceptibility show strong deviation from the Curie–Weiss behaviour as a function of temperature. Full size image Figure 2: The temperature dependence of the single-crystal magnetic susceptibility along the three principal crystalline directions. The inset shows 1/ χ for all three axes χ a , χ b and χ c . The dashed line indicates the slope of the inverse Curie–Weiss susceptibility for a paramagnet with effective moment of μ eff =1.6 μ B , close to that expected of an Ir J eff =½ state if the g -factor anisotropy is ignored. All three components of susceptibility show strong deviation from the Curie–Weiss behaviour as a function of temperature. Full size image High-temperature magnetic anisotropy As can be seen in Fig. 2 , the raw magnetic susceptibility shows a magnetic anomaly at 38 K, most likely reflecting the bipartite nature of the structure, which alleviates the magnetic frustration. Owing to the smallness of our samples and sensitivity to sample misalignment, the anisotropy at high temperatures could not be quantitatively resolved to high accuracy using superconducting quantum interference device (SQUID) magnetometry. To do so, we utilized torque magnetometry, which exclusively probes magnetic anisotropy (see discussion in Supplementary Discussion ) and is sufficiently sensitive to measure single crystals of ~10 μm dimensions. Torque magnetometry was measured by attaching an oriented single crystal to a piezoresistive micro-cantilever [13] that measures mechanical stress as the crystal flexes the lever to try to align its magnetic axes with the applied field. The mechanical strain is measured as a voltage change across a balanced Wheatstone Bridge and can detect a torque signal on the order of 10 −13 Nm. The lever only responds to a torque perpendicular to its long axis and planar surface. As a result, the orientation of the crystal on the lever (determined by X-ray measurements and the diamond-shaped morphology) defines the plane of rotation in field and which principal components of anisotropy, α ij ( i , j ε a , b , c ) are measured. To achieve this, the cantilever was mounted on a cryogenic goniometer to allow rotation of the sample with respect to magnetic field without thermal cycling. The low-temperature anisotropy was confirmed on several similar-sized single crystals. To measure α ij = χ i − χ j between 1.5 and 250 K, three discrete planes of rotation for the same crystal were used. A magnetically anisotropic material experiences a torque when its magnetization, M , is not aligned with the applied magnetic field, H , the deflection of the cantilever in a uniform magnetic field is hence a direct measure of the magnetic anisotropy, . At small fields, where the magnetic response is linear, the magnetic anisotropy is captured by a susceptibility tensor M i = χ ij H j . For an orthorhombic crystal, the magnetic axes coincide with the crystallographic directions, defining χ a , b , c . For example, for rotations in the b – c plane, the anisotropic magnetization ( M b , M c )=( χ b H b , χ c H c ) creates a torque where θ is the angle between a crystallographic axis ( c in this case) and the applied magnetic field. The geometry of the lattice is intimately connected to the magnetic anisotropy. Specifically, we note that the angle φ 0 between the honeycomb strips (see Fig. 1c ) is fixed by the geometry of the edge-shared bonding of the IrO 6 octahedra (see Fig. 3a ). For cubic octahedra cos φ 0 =1/3, namely φ 0 ≈70°, as shown in Fig. 3a . The magnetic axes can be uniquely identified from a complete angular dependence of the torque measurements, with the amplitude of the sin2 θ dependence being proportional to the magnetic anisotropy α ij . The observed magnetic axes are independent of temperature between 300 and 1.5 K. The magnetic anisotropy, shown as data points in Fig. 3b agrees well with the differences in the low-temperature susceptibility data (grey lines in Fig. 3b ). At temperatures that are high relative to the exchange interaction energy scale, we expect that only the g -factor affects the magnetic anisotropy. We find that the ratio of the anisotropic susceptibilities α ij / α jk asymptotically approach simple fractions at high temperature (above ∼ 100 K, see Fig. 3c ). Specifically, each Ir is in a threefold local planar environment with (almost) equidistant neighbours, and thus the Ir g -factor anisotropy can be captured by ascribing each honeycomb plane susceptibility component parallel, χ || and perpendicular, χ ⊥ to the plane (consider Fig. 3a ). This uniaxial local iridium environment combined with the relative orientation of the iridium planes, cos φ 0 =1/3, constrains the three components of susceptibility at high temperature to be equally spaced; 2 χ b = χ a + χ c (see Supplementary Discussion ) and the anisotropy ratios to be α ba / α ac =−½, α bc / α ac =½, α bc / α ab =1, just as we observe. This observation places constraints on the ordering of the principal components of the g -factor at all temperatures. 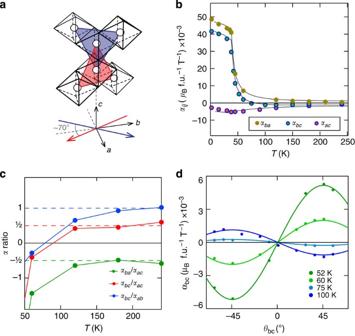Figure 3: Temperature dependence of the magnetic anisotropy. (a) Each Ir is surrounded by one of two planar, triangular environments indicated by blue and red shaded triangles, located at∼35° either side of thebaxis. (b) The anisotropy of the magnetic susceptibility as measured by torque and the differences in (SQUID) susceptibilities (grey lines) are shown as a function of temperature for all three crystallographic directions. An anomaly indicates the onset of magnetic order atTN=38 K. (c) The ratios of the anisotropic susceptibility tend to simple fractional values dictated by theg-factor anisotropy of the local planar iridium environment. (d) sin(2θ) fits to the anisotropyαbcillustrating the change of sign at∼75 K. Figure 3: Temperature dependence of the magnetic anisotropy. ( a ) Each Ir is surrounded by one of two planar, triangular environments indicated by blue and red shaded triangles, located at ∼ 35° either side of the b axis. ( b ) The anisotropy of the magnetic susceptibility as measured by torque and the differences in (SQUID) susceptibilities (grey lines) are shown as a function of temperature for all three crystallographic directions. An anomaly indicates the onset of magnetic order at T N =38 K. ( c ) The ratios of the anisotropic susceptibility tend to simple fractional values dictated by the g -factor anisotropy of the local planar iridium environment. ( d ) sin(2 θ ) fits to the anisotropy α bc illustrating the change of sign at ∼ 75 K. Full size image Reordering of the principal magnetic axes The striking reordering of the principal components of susceptibility revealed in torque and SQUID magnetometry is associated with a strong deviation from the Curie–Weiss behaviour as the temperature is lowered: α bc changes sign at T ≈75 K ( Fig. 3d ; Supplementary Figs 5 and 6 ). This is in stark contrast to spin-isotropic Heisenberg exchange systems where the low-temperature susceptibility reflects the g -factor anisotropy observed at high temperatures, even in the presence of spatially anisotropic exchange [3] . The change of sign of α bc arises because χ b softens, becoming an order of magnitude greater than χ a and ∼ 5 × χ c ( Figs 2 and 3b ). As a result, the susceptibility cannot be parameterized by a Curie–Weiss temperature: the linear extrapolation of all three components of inverse susceptibility to the temperature axis depends strongly upon the temperature range considered. Between 50 and 150 K the extrapolation of all three components of inverse susceptibility is negative, consistent with the absence of net moment in the ordered state. However, at higher temperatures (200–300 K) the inverse susceptibilities 1/ χ b ,1/ χ c extrapolate to positive temperature intercepts (see Fig. 2 ) indicating a ferromagnetic component to the interactions. Above 200 K, 1/ χ the Curie–Weiss slope gives μ e ff ≈1.6 μ B , consistent with a J eff =½ magnetism. The observed 10-fold increase in χ b cannot be driven by the g -factor of the local iridium environment, whose geometric constraints are temperature independent (see Supplementary Discussion ). The temperature dependence of χ b must therefore arise from spin–anisotropic exchange. We note that all the c -axis bonds have the Ir–O 2 –Ir plane normal to the b axis, whether they preserve or rotate between the two honeycomb orientations (see the full structure in Supplementary Figure 3A and a schematic in Fig. 4a —green shading indicates the Ir–O 2 –Ir planes). This is the only Ir–O 2 –Ir plane that is normal to a crystallographic axis. This coupling of the spin-anisotropy to the structure, provides evidence for spin–anisotropic exchange across the c -axis links, and by extension should be present in all Ir–O 2 –Ir exchange paths. This likely arises from the interfering exchange mechanism suggested by JK in the context of the Kitaev model (see Supplementary Discussion ). 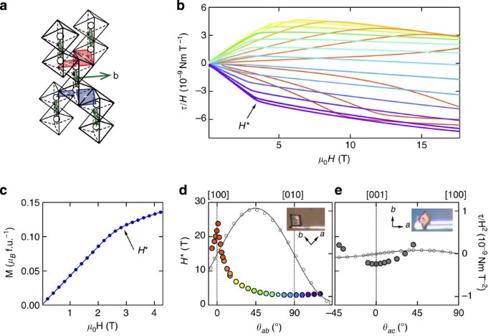Figure 4: Low-temperature magnetic properties of the ‹1›-Li2IrO3. (a) The Ir–O2–Ir planes defining three orthogonal directions of the spin-exchange, one parallel toand the other two parallel to, labelled + and − (is the unit vector alonga). This connects to the notation used to describe the Kitaev Hamiltonian inSupplementary Information III. (b) Torque signalτdivided by the applied magnetic fieldHat a temperature of 1.5 K, illustrating a linear low-field dependence and a kink atH*, which is strongly angle dependent (colours correspond to angles shown in (d)). (c) Magnetization versus magnetic field applied along thebaxis at a temperature of 15 K. (d,e) The angle dependenceθab/acof the kink fieldH* of the ordered state (full circles, left axes) with respect to the crystallographic axesa,bandc.H* is correlated to the magnetization anisotropyαij(open circles, right axes) indicating a common moment atH* in all field orientations. Figure 4: Low-temperature magnetic properties of the ‹1›-Li 2 IrO 3 . ( a ) The Ir–O 2 –Ir planes defining three orthogonal directions of the spin-exchange, one parallel to and the other two parallel to , labelled + and − ( is the unit vector along a ). This connects to the notation used to describe the Kitaev Hamiltonian in Supplementary Information III . ( b ) Torque signal τ divided by the applied magnetic field H at a temperature of 1.5 K, illustrating a linear low-field dependence and a kink at H *, which is strongly angle dependent (colours correspond to angles shown in ( d )). ( c ) Magnetization versus magnetic field applied along the b axis at a temperature of 15 K. ( d , e ) The angle dependence θ ab / ac of the kink field H * of the ordered state (full circles, left axes) with respect to the crystallographic axes a , b and c . H * is correlated to the magnetization anisotropy α ij (open circles, right axes) indicating a common moment at H * in all field orientations. Full size image Low-temperature magnetic properties The softening of χ b is truncated at 38 K by a magnetic instability. Within the ordered state, the magnetization increases linearly with applied field ( Fig. 4c , τ / H in Fig. 4b ; Supplementary Fig. 6 ). At sufficiently high magnetic fields H *, the magnetization kinks abruptly. This corresponds to an induced moment of ≈0.1 μ B . Above H *, the finite torque signal reveals that the induced moment is not co-linear with the applied field, consistent with the finite slope observed at these fields in Fig. 4c . This shows that in the phase above H * the induced magnetization along the field direction is not yet saturated (the value is well below the expected saturated Ir moment of ∼ 1 μ B for J eff =½). The angular dependence of both the slope of the linear regime and the kink field H *, exhibit an order of magnitude anisotropy with field orientation ( Fig. 4d,e ). Such strong anisotropy in a spin-½ system highlights the strong orbital character arising from the spin–orbit coupling, again in contrast to spin-½ Heisenberg anti-ferromagnetism [3] . There is a very interesting connection between the layered honeycomb Li 2 IrO 3 and the polytype studied here. The ‹1›-Li 2 IrO 3 is distinguished by its c -axis bond, which either preserves or rotates away from a given honeycomb plane (see Fig. 5a ; Supplementary Fig. 7 ); in the case that all the bonds preserve the same plane, the resulting structure is the layered honeycomb system. Further polytypes can be envisioned by tuning the c -axis extent of the honeycomb plane before switching to the other orientation (see Fig. 5b ). We denote each polytype ‹ N ›-Li 2 IrO 3 , where ‹ N › refers to the number of complete honeycomb rows (see Fig. 5b ; Supplementary Fig. 8 ), and the family as the ‘harmonic’-honeycombs, so named to invoke the periodic connection between members. The layered compound, ‹∞›-Li 2 IrO 3 (ref. 14 ) and the hypothetical hyper-honeycomb structure, ‹0›-Li 2 IrO 3 (ref. 15 ) are the end members of this family (see also Supplementary Information IV ). The edge-sharing geometry of the octahedra preserves the essential ingredients of the Kitaev model and this is universal for this family of polytypes. Each structure is a material candidate for the realization of a three-dimensional spin liquid in the pure Kitaev limit (see Supplementary Discussion and for ‹0›-Li 2 IrO 3 see refs 15 , 16 , 17 ). 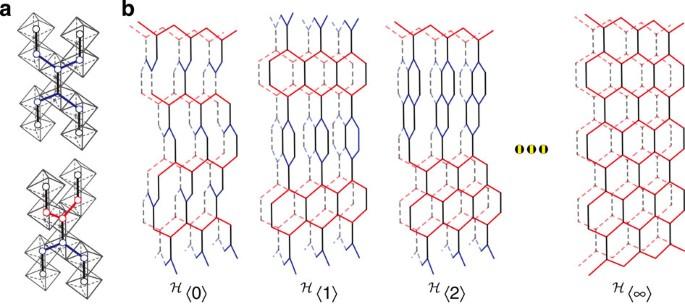Figure 5: Introducing the harmonic honeycomb series. (a) Two kinds ofc-axis bonds (black links) in the harmonic honeycomb family ‹N›-Li2IrO3are shown, one linking within a honeycomb plane (for example blue to blue, top) and one that rotates between honeycomb planes (for example red to blue, bottom). For undistorted octahedra, these links are locally indistinguishable, as can be observed by the local coordination of any Ir atom (also seeFig. 3a). (b) These building blocks can be used to construct a series of structures. The end members include the theoreticalN=0 ‘hyper-honeycomb’15,16,17and theN=∞ layered honeycomb14. HereNcounts the number of complete honeycomb rows in a section along thecaxis before the orientation of the honeycomb plane switches. Figure 5: Introducing the harmonic honeycomb series. ( a ) Two kinds of c -axis bonds (black links) in the harmonic honeycomb family ‹ N ›-Li 2 IrO 3 are shown, one linking within a honeycomb plane (for example blue to blue, top) and one that rotates between honeycomb planes (for example red to blue, bottom). For undistorted octahedra, these links are locally indistinguishable, as can be observed by the local coordination of any Ir atom (also see Fig. 3a ). ( b ) These building blocks can be used to construct a series of structures. The end members include the theoretical N =0 ‘hyper-honeycomb’ [15] , [16] , [17] and the N =∞ layered honeycomb [14] . Here N counts the number of complete honeycomb rows in a section along the c axis before the orientation of the honeycomb plane switches. Full size image Finally, we speculate on the consequences and feasibility of making other members of the ‹ N ›-Li 2 IrO 3 family. Both the layered ‹∞›-Li 2 IrO 3 and the ‹1›-Li 2 IrO 3 are stable structures, implying that intermediate members may be possible under appropriate synthesis conditions. The building blocks shown in Fig. 5a connect each member of the harmonic honeycomb series in a manner that is analogous to how corner-sharing octahedra connect to the Ruddlesden–Popper (RP) series. Indeed, despite the fact that members of the RP family are locally identical in structure, they exhibit a rich variety of exotic electronic states, including superconductivity and ferromagnetism in the ruthenates [18] , [19] , multiferroic behaviour in the titanates [20] , collosal magnetoresistance in the manganites [21] and high-temperature superconductivity in the cuprates [22] . The harmonic honeycomb family is a honeycomb analogue of the RP series, and its successful synthesis could similarly create a new frontier in the exploration of strong spin–orbit-coupled Mott insulators. Synthesis Powders of IrO 2 (99.99% purity, Alfa-Aesar) and Li 2 CO 3 (99.9% purity, Alfa-Aesar) in the ratio of 1:1.05, were reacted at 1,000 °C, then reground and pelletized, taken to 1,100 °C and cooled slowly down to 800 °C. The resulting pellet was then melted in LiOH in the ratio of 1:100 between 700 and 800 °C and cooled at 5 °C per hour to yield single crystals of ‹1›-Li 2 IrO 3 . The crystals were then mechanically extracted from the growth. Single-crystal X-ray refinements were performed using a Mo-source Oxford Diffraction Supernova diffractometer.Please see Supplementary Discussion for a detailed analysis. Magnetic measurements Two complementary techniques were used to measure the magnetic response of single crystals of ‹1›-Li 2 IrO 3 ; a SQUID magnetometer was employed to measure magnetization and a piezoresistive cantilever to directly measure the magnetic anisotropy. The magnetization measurements were performed in a Cryogenic S700X. Owing to the size of the single crystals, the high-temperature magnetization was near the noise floor of the experiment. Nevertheless, SQUID-measured anisotropies at high temperatures were close to those measured by torque, with absolute values of χ a (300 K)=0.0021 μ B T −1 f.u. and χ b =0.0024 μ B T −1 f.u. Curie–Weiss fits to the linear portion of the susceptibility yielded an effective moment of μ eff =1.6(1)μ B , consistent with J eff =½ magnetism. However, the SQUID resolution was not adequate to determine the susceptibilities anisotropy at high temperature to the accuracy we required (see Fig. 2 ). To resolve the magnetic anisotropy throughout the entire temperature range, we employed torque magnetometry, where a single crystal could be precisely oriented. Although the piezoresistive cantilever technique is sensitive enough to resolve the anisotropy of a ∼ 50 μm 3 single crystal, and hence ordering of susceptibilities at high temperature, the absolute calibration of the piezoresistive response of the lever leads to a larger systematic error than in the absolute value of the susceptibility measured using the SQUID at low temperature. To reconcile these systematic deficiencies in both techniques, the torque data were scaled by a single common factor of the order of unity, for all field orientations and temperatures, so as to give the best agreement with the differences between the low-temperature susceptibilities as measured using the SQUID. The rescaled torque data were thus used to resolve the magnetic anisotropy at high temperature where the susceptibility is smallest. Torque magnetometry was measured on a 50 × 100 × 40 μm 3 single crystal (5.95 × 10 −9 mol Ir) employing a piezoresistive micro-cantilever [13] that measures mechanical stress as the crystal flexes the lever to try to align its magnetic axes with the applied field. The mechanical strain is measured as a voltage change across a balanced Wheatstone Bridge and can detect a torque signal on the order of 10 −13 Nm. Torque magnetometry is an extremely sensitive technique and is well suited for measuring very small single crystals. The cantilever was mounted on a cryogenic goniometer to allow rotation of the sample with respect to magnetic field without thermal cycling. The lever only responds to a torque perpendicular to it’s long axis and planar surface, such that the orientation of the crystal on the lever and the plane of rotation in field could be chosen to measure the principal components of anisotropy, α ij . The low-temperature anisotropy was confirmed on several similar-sized single crystals. However, to measure α ij = χ i − χ j between 1.5 and 250 K, three discrete planes of rotation for the same crystal were used. When remounting the sample to change the plane of rotation, care was taken to maintain the same center of mass position of the crystal on the lever to minimize systematic changes in sensitivity. Magnetic fields were applied using a 20-T superconducting solenoid and a 35-T resistive solenoid at the National High Magnetic Field Laboratory, Tallahassee, FL. How to cite this article: Modic, K. A. et al. Realization of a three-dimensional spin–anisotropic harmonic honeycomb iridate. Nat. Commun. 5:4203 doi: 10.1038/ncomms5203 (2014).